Why nanotubes grow chiral Carbon nanotubes hold enormous technological promise. It can only be harnessed if one controls their chirality, the feature of the tubular carbon topology that governs all the properties of nanotubes—electronic, optical, mechanical. Experiments in catalytic growth over the last decade have repeatedly revealed a puzzling strong preference towards minimally chiral (near-armchair) tubes, challenging any existing hypotheses and making chirality control ever more tantalizing, yet leaving its understanding elusive. Here we combine the nanotube/catalyst interface thermodynamics with the kinetic growth theory to show that the unusual near-armchair peaks emerge from the two antagonistic trends at the interface: energetic preference towards achiral versus the faster growth kinetics of chiral nanotubes. This narrow distribution is inherently related to the peaked behaviour of a simple function, xe −x . The broad interest in carbon nanotubes (CNTs), unceasing since their first clear observation [1] , has been fuelled by possible technological applications derived from their unique fundamental properties [2] , [3] , [4] . All of the latter are in turn determined by the helical fashion of folding a tube, specified by the chiral angle χ between its circumference and the zigzag motif in the honeycomb lattice of atoms, with χ =0 and χ =30° for the achiral types, zigzag and armchair. Alternatively, a pair of chiral indices ( n , m ) is commonly used, the integer components of the circumference vector [2] . In spite of such a defining role of chirality, most synthetic methods yield a broad distribution with mixed properties. To achieve control of the CNT type remains a great challenge; what physical mechanisms determine the chirality distribution and even why the nanotubes grow chiral is still unsettled. Although the discovery paper by Iijima [1] has already suggested one key, connecting the tube ability to grow with the kinks at its end and the screw dislocation model, it took almost two decades until the first equation [5] related the speed of growth and chirality, R ~sin χ . It should further be useful to think, in hindsight, of the probable causes of such a delay. Besides the difficulties of determining chirality in experiments, in theory it was ambiguous as to whether the chiral angle must be measured from the zigzag (as χ ) or perhaps from the armchair (as χ − ≡ 30°− χ ) direction. While each choice appears valid from a pure symmetry standpoint, their kinetic predictions are opposite (with one favouring armchair and the other, zigzag CNTs), and thus one stumbles upon an immediate contradiction. Another diversion was due to a simple thermodynamic argument that the lower energy of the tube edge, rather than its kinetic advantage of having kinks, must determine the dominant CNT type, pointing towards the armchair tubes, especially (10,10) broadly discussed by Smalley et al. [6] This situation, together with recent advances in synthesis featuring, in several cases, very narrow chiral distributions [7] , [8] , [9] , poses a compelling question as to which factors—thermodynamic preference to lower energy, or kinetic preference of higher speed—play a major role in defining the distribution of CNT product. The true answer appears to be ‘both’, and the analysis below shows how the subtle interplay of these physical factors defines the more probable chirality choices. In particular, it explains why at lower temperatures on solid catalyst particles the yield peaks near armchair types ( n , n –1), never exactly armchair, although quite close. The evolution of chemical vapour deposition (CVD) techniques and chirality characterization methods [10] has led to improvements in chiral selectivity [7] , [8] , [9] , [11] , [12] , [13] , [14] , [15] , [16] , eventually reaching >50% fraction for a single-CNT type and ~90% for semiconducting tubes [9] . More intuitive strategies such as post-growth selection [17] , [18] , rational synthesis [19] , [20] , [21] , or seeding [22] , [23] , [24] do, in principle, offer great selectivity but lack the scalability of CVD. Further improvements of the latter direct synthesis techniques thus call for better understanding of the growth process. Yet, its mechanism and especially the causes behind its occasional success in chiral preference remain puzzling. In modelling efforts [25] , direct molecular dynamics (MD) or Monte Carlo simulations, although invaluable in many respects, generally fail to produce nondefective CNT structures of a well-defined diameter and recognizable chirality, regardless of the precision of interatomic potentials—from classical [26] , [27] , [28] , [29] to tight-binding [30] , [31] and density functional theory (DFT) [32] . This is caused by the short accessible timescale due to sheer computational limitations. Alternating MD with Monte Carlo relaxation has produced ‘definable’ [33] but occasionally changing [34] chirality. It is clear that a physical theory bridging the gap between atomistic dynamics and macroscopic scales is needed to interpret both the experiments and simulations. In the present work, we propose a theory that reconciles the kinetic and thermodynamic arguments within a unified model. We show how the rigid state of the catalyst causes the two factors to exhibit opposite trends, where nucleation energetics penalizes chiral CNTs while growth rate penalizes achiral tubes. These two trends find a ‘compromise’ in minimally chiral CNTs, which explains why these peculiar types, such as (6,5), are robustly observed in many experiments. CNT abundance We treat the CNT abundance by type as the result of the action of two main factors. At proper conditions, the nanotubes nucleation occurs, with probability N n , m of certain chiral type. It is followed by the steady carbon accretion by each tube, with its growth rate R n , m . After some time, the fraction of the tubes of chirality ( n , m ), that is, their relative abundance A n , m in the accumulated material, is determined by the product of both these factors [35] , as A n , m = N n , m · R n , m (see Supplementary Note 1 for a more general analysis). Instead of the chiral indices, using the tube diameter d and chiral angle χ gives A ( χ , d )= N ( χ , d )· R ( χ , d ). Below we explore the physical mechanisms defining the right-hand side, in particular the case of a solid catalyst with a rigid shape, which yields sharp chiral angle selectivity in A ( χ , d ), as empirical evidence suggests. Continuum model Before discussing the details of atomistic study, it is useful to explore the key ideas in terms of simpler continuum model, which not only offers valuable insight but is even able to make accurate overall predictions. During nucleation, as carbon atoms attach to a nascent CNT nucleus, adding new hexagonal and pentagonal rings to it, the chirality of a CNT becomes permanently ‘locked in’ when the final 6th pentagon is added to the hemispherical cap (barring further changes of CNT type if pentagon–heptagon defects form at the edge, which is generally a rare event [36] ). From this six-pentagon nucleus a cylindrical CNT structure can further grow by adding only hexagons, in a periodic fashion. The free energy of the critical nucleus contains two contributions, G *= G cap +Γ. The first one, G cap , originates from the ‘elastic’ energy of cap per se and does not depend on χ (ref. 37 ). The second term Γ represents the contact interface between the sp 2 -carbon lattice edge and the metal catalyst, and does contain chirality dependence since the edge energy γ ( χ ) varies with the crystallographic orientation and Γ( χ , d ) ≡ πdγ ( χ ). Whereas previous studies on edge energetics [38] assumed either vacuum or a liquid-like catalyst that fully adapts to the edge profile, chiral-selective CVD growth is usually reported at comparatively low temperatures [8] , [9] when the catalyst particle is solid [9] . Accordingly, the metal side of the interface is rather a rigid atomic plane, and the structure of this interface affects both the energy of the nucleus and the subsequent insertion of new C atoms during growth. In Fig. 1 inset, the CNT is in contact with the catalyst which is represented locally as a continuous plane corresponding to an atomic terrace in a solid particle. The catalyst particle surface does not have to be planar. Since the important region is the narrow ring of CNT–catalyst contact, even a single atomic terrace running around the particle circumference will act essentially equivalent to a plane. The CNT is also continuous, but the kinks along its edge are retained according to the tube chirality, Fig. 1a–c . These kinks cause the gaps between the substrate and the CNT, shown in Fig. 1b,c for ( n ,3) and ( n ,1) tubes, with an associated energy penalty, relative to the tight contact in case of achiral tube in Fig. 1a . For the hexagonal lattice of CNT, the two fundamental achiral edges—armchair ( A ) and zigzag ( Z )—form tight low-energy contacts. The interface energy for chiral tubes is higher, roughly in proportion with the number of kinks, which increases linearly with χ for near- Z tubes, or with χ − for near- A tubes. In other words, γ ( x )≈ γ + γ ′ ·x , where x is the angular deviation from the achiral direction: near the Z -type x = χ , γ = γ Z ≡ γ (0), and γ ′=∂ γ /∂ χ | χ =0 , or near the A -type x = χ − , γ = γ A ≡ γ (30°), and γ ′=−∂ γ /∂ χ | χ =30° . 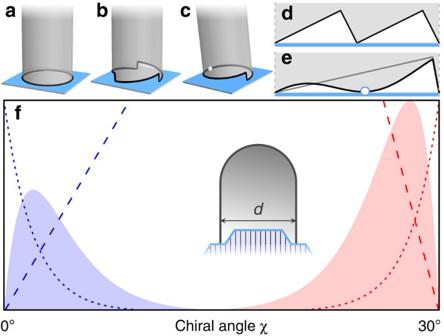Figure 1: Continuum model of the CNT–catalyst system. Schematic representation of: (a) achiral; (b) multiple-kink chiral; and (c) single-kink chiral CNTs on a flat substrate. Unrolled CNT–substrate interfaces for (d) two-kink and (e) single-kink nanotubes show the nanotube tilt off the vertical, reducing the edge-substrate gap; the white dot incandemarks the contact point. The abundance distributionsA(χ)~χ e−χcomputed as the product of nucleation (dotted) and growth rate (dashed) terms are shown inffor near-Z(blue) and near-A(red) chiralities. The inset illustrates a nascent CNT of diameterdon a solid catalyst. Figure 1: Continuum model of the CNT–catalyst system. Schematic representation of: ( a ) achiral; ( b ) multiple-kink chiral; and ( c ) single-kink chiral CNTs on a flat substrate. Unrolled CNT–substrate interfaces for ( d ) two-kink and ( e ) single-kink nanotubes show the nanotube tilt off the vertical, reducing the edge-substrate gap; the white dot in c and e marks the contact point. The abundance distributions A ( χ )~ χ e − χ computed as the product of nucleation (dotted) and growth rate (dashed) terms are shown in f for near- Z (blue) and near- A (red) chiralities. The inset illustrates a nascent CNT of diameter d on a solid catalyst. Full size image Since γ ( χ ) is largest in the intermediate range of χ ≈15°, such tubes are unlikely to nucleate, and one should focus on just the neighbourhoods of Z and A chiralities. Then we write: The essential result here is that the nucleation probability falls rapidly as e − β · x with chiral angle x , and β = πdγ′/k B T . A distinction for single-kink cylinders, representing the nanotubes ( n ,1) and ( n , n –1), should be noted. Their symmetry allows them to tilt off the vertical axis, improving the interface contact. Figure 1d,e illustrates it by ‘unrolling’ the CNT–substrate interface area for two-kink and single-kink tubes. In the latter case, the effect of tilt leads to a reduction of the tube-substrate separation, appearing as a sinusoid along the circumference as shown in Fig. 1e , enabling a substantial closure of the gap between substrate and tube edge, recovering up to as much as 70% of the energy penalty—see Supplementary Fig. 1 and Supplementary Note 2 . For the growth rate term R ( χ , d ), we augment the screw dislocation model [5] by including the kinks created by thermal fluctuations on A and Z edges [39] , and accounting for the energy penalty ~1/ d 2 from the wall curvature. In the liquid-catalyst model, when the metal adapts to the CNT edge with a one-to-one termination, calculations suggest that the cost E A to create a pair of kinks on an A edge is zero, and consequently [5] R ∝ χ . However, on a solid surface, creating a pair of kinks destroys the perfect contact between the CNT and substrate, costing energy. Therefore E A has a noticeable magnitude, and the dependence becomes bimodal with minima at the A and Z ends of the chiral angle range, and a maximum at the 19.1° magic angle [39] , [40] of (2 m , m ) tubes. The final expression, linearized near the A and Z bounds of chirality, reads as follows, where C =3.9 eV Å 2 per atom is the bending rigidity of graphene [41] . The term x in parentheses corresponds to the density of geometry-imposed kinks, proportional to the vicinal-edge angular deviation from the main achiral direction, and the term (typically small) represents the additional fluctuational kinks. The free-energy barriers for the initiation of a new atomic row on A or Z edge are E = E Z near the Z -type where , or E = E A near the A -type where x = χ − . Multiplying together the nucleation and growth terms presents the key to understanding the observed selectivity for near- A chiralities [9] . At a given diameter, a function with a sharp peak near zero (or near 30°). This is the essential result of our continuum consideration. Figure 1f illustrates this peaked distribution character. The two distributions for near- Z (blue) and near- A (red) chiral angles are plotted assuming equal interface energies and growth barriers: γ A = γ Z , E A = E Z . However, if either A or Z has a lower energy, the opposite peak distribution is additionally penalized by , with ΔΓ=Γ Z −Γ A on the order of eV, and then one would expect to observe only one side of the distribution. These continuum-model predictions turn out to be remarkably robust. To see this, below we present the atomistic calculations of the relevant quantities, and proceed to simulate example CNT-type distributions. Atomistic model Computations were performed using a flat Ni(111) slab to represent the solid catalyst. We used a classical force-field MD sampling complemented with static DFT computations (on Ni and also Co slabs), as detailed in Methods. To investigate the chiral selectivity of nucleation, two sets of CNTs are chosen, with d ≈0.8 and 1.2 nm, to include the prominent in experiments (6,5) [9] and (9,8) [8] CNTs. 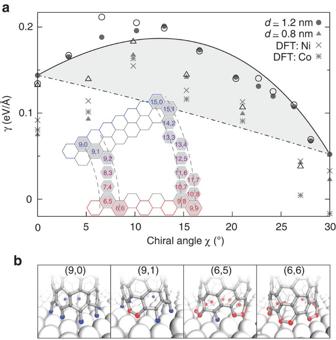Figure 2: Chirality-dependent CNT–catalyst contact energies, governing the nucleation. (a) Interface energies calculated with MD (circles and triangles) and fitted with analytical expression (solid line) for two CNT sets (inset; dashed arcs denote the range of diameter variation in each set). Static DFT calculations on Ni and Co are also shown. Open and filled symbols denote regular (hexagonal) and KleinZ-edge structures—see sample atomistic structures inb. The dash-dotted line, calculated asγ(χ)=2γAsinχ+2γZsin (30°−χ),38corresponds to liquid-catalyst case. Inb, the blue and red atoms highlight theZandAedges, respectively. Figure 2a shows the calculated CNT–substrate interface energies. The atomistic structures for the (9,0), (6,5), and (6,6) CNTs are shown in Fig. 2b , where the tilting of the (6,5) and (9,1) CNT to reduce the interface energy is seen clearly. We found that for the smaller-diameter set, for near- Z edges the Klein structure, in which a normal zigzag edge has an extra C atom (blue in Fig. 2b ) attached to each hexagon [42] , is favored over the standard closed-hexagons, whereas the larger-diameter set shows little preference either way. All data display the same qualitative behaviour conforming to the above discussion, and are generally in good quantitative agreement. Both bounds of the chiral angle range (achiral CNTs) are energy minima, and the energy is higher for Z than for A tubes. The curves show the fit of γ ( χ ) using the analytical expression from earlier work [38] for solid- and liquid-like cases. Figure 2: Chirality-dependent CNT–catalyst contact energies, governing the nucleation. ( a ) Interface energies calculated with MD (circles and triangles) and fitted with analytical expression (solid line) for two CNT sets (inset; dashed arcs denote the range of diameter variation in each set). Static DFT calculations on Ni and Co are also shown. Open and filled symbols denote regular (hexagonal) and Klein Z -edge structures—see sample atomistic structures in b . The dash-dotted line, calculated as γ ( χ )=2 γ A sin χ +2 γ Z sin (30°− χ ), [38] corresponds to liquid-catalyst case. In b , the blue and red atoms highlight the Z and A edges, respectively. Full size image Our computations pertaining to the growth kinetics are summarized in Fig. 3 . We build upon our earlier approach for graphene [39] , adapting it for the case of CNTs. 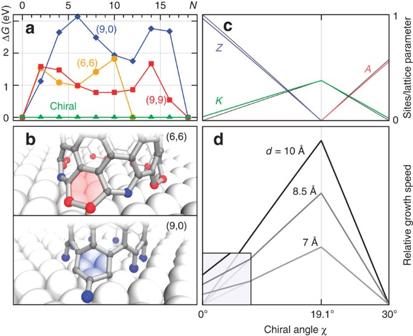Figure 3: Chirality-dependent growth rate of CNTs. (a) Free-energy profiles during the growth of a new ring of hexagons on (red, orange)Aand (blue)Zedges as a function of number of added atomsN. The green line corresponds to barrierless chiral-edge growth. (b) The atomic configurations after first dimer addition,N=2. (c) Linear density of different site types on CNT edges as a function of chiral angle. (d) The resulting CNT growth rate as a function of chiral angle for several diameters (inset shows the effect of thermal kinks). Figure 3a shows the energy changes with the addition of a new row of carbon atoms, dimer by dimer, for (6,6), (9,9) and (9,0) CNTs (see also Supplementary Figs 2 and 3 and Supplementary Note 3 for activation barrier calculations, showing the same trends). All three curves depart from the ‘nucleation to kink-flow’ scenario of graphene, the reason being the constantly changing tilt angle of the CNTs. However, both A curves (red, orange) show essentially the same height for the first dimer addition and the same maximum height (closer to the end). The Z curve bears the same qualitative character, having an initial and a final maximum. The system cycles through the curve with every new full ring of hexagons, after which Δ G returns to 0. The maximum height of each curve determines the free-energy barrier that needs to be overcome for successful addition of each new row of hexagons, Δ G A ≈1.67−1.86 eV and Δ G Z >3 eV (calculations for the (9,0) CNT yield multiple intermediate structures with topological defects of energies lower than perfect hexagonal structures, an additional complication for Z -CNT growth). These are the terms that penalize the pure A and Z tubes, compared with the chiral ones (green line in Fig. 3a ), by an additional factor and thus effectively remove them from the product distribution, despite their favourable cap-nucleation energies. The atomic configurations for the first dimer addition to the (6,6) and (9,0) CNTs are shown in Fig. 3b . Figure 3c shows the concentrations of different site types— Z , A and K (kink)—as a function of χ [38] , [39] , [40] . Thin black lines show the intrinsic, topologically required values. Finally, Fig. 3d shows the CNT growth speed. Higher temperatures favour kink formation and promote the growth of zigzag and armchair CNTs. However, under realistic conditions, when k B T ≪ Δ G , the growth rate of achiral CNTs is negligible. Among different diameters d , the curvature of the wall penalizes insertion of C atoms into small-diameter CNTs, as in equation (2). Figure 3: Chirality-dependent growth rate of CNTs. ( a ) Free-energy profiles during the growth of a new ring of hexagons on (red, orange) A and (blue) Z edges as a function of number of added atoms N . The green line corresponds to barrierless chiral-edge growth. ( b ) The atomic configurations after first dimer addition, N =2. ( c ) Linear density of different site types on CNT edges as a function of chiral angle. ( d ) The resulting CNT growth rate as a function of chiral angle for several diameters (inset shows the effect of thermal kinks). Full size image We now have all the ingredients to calculate the relative abundance of different CNT types from atomistic computations. The distributions for the two CNT data sets in Fig. 4a both show a strong predominance of ( n , n –1) near-armchair CNTs. The selectivity of distributions is actually so strong that one has to increase the temperature to T =2700 K when plotting these distributions; at T =900 K, both show effectively single peaks for (6,5) or (9,8) CNTs. Further, one can use either data set to compute a general ( n , m ) distribution through interface energy fitting. An example is shown in Fig. 4b . The peak in diameter distribution results from the competition between the interface energy, favoring smaller d in equation (1), and a prefactor due to the configurational entropy of CNT caps [37] , [43] , favoring larger diameters [2] , which scales approximately [44] as ~ d 8 (details in Supplementary Note 4 ). In a real CVD experiment, there will be additional constraints on d from the size of catalyst particles. Then the product distribution will be a slice of Fig. 4b with prominent ( n , n –1) peaks, such as those shown in Fig. 4a . 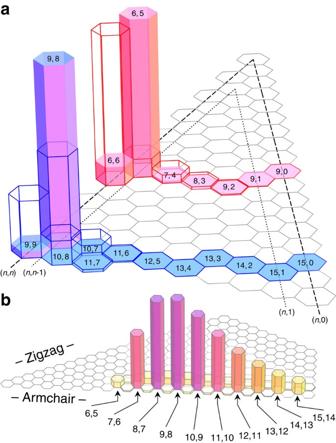Figure 4: Predicted CNT-type distributions. (a) Distributions calculated directly based on atomistic computations for two CNT sets (d≈0.8 nm and 1.2 nm, each distribution is normalized separately). The empty bars show chirality distributions for liquid-catalyst case. (b) Full (n,m) distribution based on an analytical fit to MD interface energies. For all plots, the temperature was artificially set to about three times the typical experimental value to make the heights visible. Figure 4: Predicted CNT-type distributions. ( a ) Distributions calculated directly based on atomistic computations for two CNT sets ( d≈ 0.8 nm and 1.2 nm, each distribution is normalized separately). The empty bars show chirality distributions for liquid-catalyst case. ( b ) Full ( n , m ) distribution based on an analytical fit to MD interface energies. For all plots, the temperature was artificially set to about three times the typical experimental value to make the heights visible. Full size image By similar logic, our theory suggests a possibility to highly selectively achieve the near- Z ( n ,1) CNTs, if a catalyst favors Z interface over A . While ( n , n –1) are always semiconducting, the ( n ,1) series contains all three CNT families (metallic and two semiconducting). Then, control of diameter would allow a selective synthesis of CNTs of either conductivity type. Moreover, when speculating on a possibility of catalyst–template exactly matching a certain ( n , m ) tube, we learn here that this would more likely favour the one-index-off tubes such as ( n , m ±1), to allow for rapid kinetics at the cost of somewhat higher energy of the contact and nucleation. If however, the tight contact is dominant— γ ′ in equation (1) is large—the previously neglected term of equation (2) permits a non-zero growth rate even for perfectly matching tube–catalyst combinations ( x =0), for example, armchair on flat substrate. This way catalyst matching can offer direct chirality control, though perhaps at a significantly reduced rate/yield. We can also compare the simulated distributions with a liquid-catalyst model (dash-dotted line in Fig. 2a and the kink formation energy [5] E A =0). The results are shown in Fig. 4a as hollow bars and display much greater presence of armchair CNTs in the overall broader distribution. In reality, irregular and highly mobile structure of a liquid catalyst may flatten the energy landscape in Fig. 2a and thus further broaden the distribution, making the kinetic route of selection dominant. If E A >0, the fastest-growing tubes have χ =19.1° ( Fig. 3d ), which corresponds to (2 m , m ) CNTs. Finally, with χ -unbiased nucleation probability and E A →0, one recovers the proportionality result [5] , A ∝ χ . We also note that additional flexibility could potentially be gained by performing the nucleation and steady-state growth stages under different conditions such as catalyst state, for example, nucleation on solid followed by growth on liquid should favour achiral types. In summary, we discovered that the origins of chirality can only be understood if the kinetic and thermodynamic aspects of CNT growth are considered concurrently. The growth kinetics is aided by the kinks at the tube edge and thus favours the chiral types, in proportion to their chiral angle. The thermodynamic nucleation barrier, on a solid catalyst, is lower for the kinkless edges of achiral tubes. In spite of complex and random variability of numerous atomic structures in the process, the overall product abundance can be summed up in a remarkably compact mathematical expression: xe − β · x . For lower temperatures and a solid catalyst, this function has a sharp maximum near zero, which explains the observations of near-armchair nanotubes in experiments. Higher T and a liquid catalyst make contact energies effectively equal ( β →0) and nucleation of various types similarly probable, with the abundance then nearly proportional to chiral angle. This demonstrates that the approach is sufficiently comprehensive, being able to explain rather disparate facts accumulated over decades of experiments, from broader chiral distributions to very narrow, almost single-type peaks. Furthermore, we believe that the newly gained insight may enable finding ways to engineer chiral-selective nanotube production, thus advancing a variety of long-awaited applications, all pending availability of properly pure material. Note added in proof : While this paper was under consideration a study was published showing extremely strong preference for a specific CNT type that its authors attribute to catalyst-matching [45] . In terms of equation (1) this translates into a large magnitude of γ ′. The authors of an even more recent study [46] were able to achieve single-type selectivity via seeded growth (effectively, N n,m = δ n, 6 δ m, 6 ). In both cases, according to equations (1) and (2), the smallness of the factor which provides for the growth of catalyst-matching CNTs should result in slow growth rates/low yield. MD simulations MD sampling was performed using the canonical ( NVT ) ensemble with the ReaxFF force field [47] , [48] as implemented in the LAMMPS [49] , [50] simulation package. The basic structural properties and energetics of graphene and Ni bulk and low-index surfaces using this setup were validated in earlier work [51] . The catalyst/support is represented by a four-layer Ni(111) slab of approximately square shape and area of 90 surface unit cells (~2.3 × 2.3 nm 2 ). In all runs, the atomic motion of the bottom Ni layer is constrained to the (111) plane. Initially, a 100-ps NPT trajectory is generated, employing a Nosé–Hoover thermostat and barostat to maintain temperature T =900 K (damping parameter τ T =0.1 ps; constrained bottom-layer degrees of freedom excluded from T calculation/control), and lateral pressure tensor components P || =0 (τ P =1 ps), preserving the lateral simulation box shape. The average box sizes determined from this trajectory are used in all subsequent canonical ( NVT ) trajectories at the same temperature. All calculations use 0.25 fs timestep and ensemble averaging is obtained from 1.2 ns trajectories. DFT calculations The DFT calculations were performed with the local spin density approximation using the QUANTUM ESPRESSO package [52] . Vanderbilt ultrasoft pseudopotentials [53] were used with a plane-wave basis set cutoff of 50 Ry. The model systems consisted of a (6 × 6) Ni(111) (or Co(111)) slab supercell with three atomic layers of Ni (or Co). The positions of the bottom atomic layer were frozen during geometry optimization. The CNTs were represented by fragments two hexagons tall (60–72 C atoms) with the top edge passivated by hydrogen atoms. Correction to the ReaxFF-calculated interface energies In our previous research, we found that classical potentials including the ReaxFF parameter set employed herein yield the ratio of Z- to A -edge energies in vacuum different from the DFT result [38] , [54] . Since using ab initio MD to compute all quantities necessary for this study would be orders of magnitude beyond the available computational power, we instead utilized a ‘DFT correction’ scheme for ReaxFF. First, we computed the interface energies for the small-diameter CNT set with DFT. The relaxed structures were then used as input for ReaxFF optimization. Then we used ReaxFF to search for the global-minimum adsorbed configuration by taking a CNT fragment and sampling the rotations about the vertical axis in the 0–180° interval in steps of 5°. For each initial geometry, a low-temperature annealing is performed for 5 ps. The lowest-energy configurations were then again optimized with DFT. Thus, we obtain two data points for the DFT–ReaxFF energy difference for each CNT. This set was fitted with a πd ( A − Bχ ) model, with A and B fitting parameters, and the resulting fit used to ‘reconstruct’ the interface energies from ReaxFF simulations. The mean and median residuals of the fit were only 0.1 eV Å −1 and 0.06 eV Å −1 , respectively. It should be stressed that these differences correspond not to the same instantaneous configurations, but rather, to the closest local minima between the methods. How to cite this article: Artyukhov, V. I. et al. Why nanotubes grow chiral. Nat. Commun. 5:4892 doi: 10.1038/ncomms5892 (2014).